Physiological and genomic features of highly alkaliphilic hydrogen-utilizingBetaproteobacteriafrom a continental serpentinizing site Serpentinization, or the aqueous alteration of ultramafic rocks, results in challenging environments for life in continental sites due to the combination of extremely high pH, low salinity and lack of obvious electron acceptors and carbon sources. Nevertheless, certain Betaproteobacteria have been frequently observed in such environments. Here we describe physiological and genomic features of three related Betaproteobacterial strains isolated from highly alkaline (pH 11.6) serpentinizing springs at The Cedars, California. All three strains are obligate alkaliphiles with an optimum for growth at pH 11 and are capable of autotrophic growth with hydrogen, calcium carbonate and oxygen. The three strains exhibit differences, however, regarding the utilization of organic carbon and electron acceptors. Their global distribution and physiological, genomic and transcriptomic characteristics indicate that the strains are adapted to the alkaline and calcium-rich environments represented by the terrestrial serpentinizing ecosystems. We propose placing these strains in a new genus ‘ Serpentinomonas ’. Serpentinization is an aqueous alteration process in which low-silica ultramafic rocks (for example, olivines and pyroxenes) are oxidized and hydrolyzed with water into serpentinite, brucite, magnetite and other minerals. During these reactions, abundant hydrogen gas is produced creating the conditions capable of the abiotic reduction of carbon to produce hydrocarbons [1] . Meanwhile, during the breakdown of clinopyroxene (for example, diopside) in the serpentinization reactions, the high concentration of dissolved Ca 2+ in the serpentinizing fluid is accommodated by OH − production due to the absence of a stable Ca mineral [2] . On exposure to air at terrestrial or seawater, the Ca 2+ in the alkaline fluid reacts with dissolved inorganic carbon (DIC) [3] , [4] , [5] resulting in the precipitation of calcite at the air or seawater/serpentinizing water interfaces. Thus, the fluid issuing from the serpentinite-hosted rocks is generally highly basic, highly reduced, rich in hydrogen, methane and Ca 2+ , and poor in DIC. Serpentinization can occur at tectonic plate boundaries where the earth’s mantle is uplifted into the crustal zone and exposed to water. Before the differentiation of the lithosphere on early Earth, serpentinization was considered to be widespread in the ocean [1] . On the modern earth, active serpentinization is common in deep ocean environments, including the Mid Atlantic Ridge [6] and Mariana Forearc [7] , and is known a number of terrestrial sites: for example, California [3] , [8] , Portugal [9] , Canada [4] , Turkey [10] , Oman [11] , Italy [12] , Yugoslavia [11] , Philippines [13] and the Precambrian Shield in Finland [14] . ‘The Cedars’, located near the Russian River in northern California within the Franciscan Subduction Complex, is an active terrestrial serpentinizing site [3] , [8] . The springs in The Cedars discharge from rocks emplaced during the middle Jurassic (~\n170 Ma) [15] . The spring waters discharging from The Cedars ultra-mafics have very high pH values (~\n11.6), low Eh values (~\n−500 mV or less) and a relatively high concentration of Ca 2+ (~\n1 mM) [3] . In addition, the spring waters are meteoric in origin, with low concentrations of dissolved organic carbon (DOC), sodium and potassium, and undetectable levels of ammonium, phosphate and electron acceptors (dissolved oxygen, nitrate and sulphate) [3] ; a combination that is very challenging for life. For instance, while there is plenty of energy (electron donor) in the form of hydrogen produced by serpentinization, there are very low levels of electron acceptors as well as low levels of protons and sodium to be used for establishing a membrane potential (cation motive force). In addition, DOC is also limited [3] and the soluble form of carbon dioxide at pH 11 and above is primarily the carbonate ion (CO 3 2− ), which is considered to be an unavailable form of DIC for microbes. Therefore, according to present day paradigms of metabolism, it is very difficult to explain how to make a living with regard to performing respiration, carbon assimilation, pumping protons or sodium for energy metabolism and cytoplasm homeostasis in The Cedars springs. The Cedar springs are fed by either or both of two different hyper alkaline serpentinizing groundwaters (shallow and deep) that have different geochemical properties [3] , and the microbial communities of these springs were found to be strongly correlated with the source groundwater feeding them [16] . While the shallow groundwater communities were similar to those described in other terrestrial serpentinizing sites, the deep groundwater microbial community was distinctly different from any other previously described terrestrial serpentinizing community [16] . The shallow groundwater-fed springs were numerically dominated by microbes related to the genus Hydrogenophaga within Betaproteobacteria [16] . Furthermore, alkaline fluid from other terrestrial serpentine-hosted ecosystems also contained abundant Hydrogenophaga -related microbes [17] , [18] , [19] , [20] . Therefore, these microbes appear to be well adapted to geochemical settings occurring at the continental serpentinizing sites, distinguishing them from other cultivated Hydrogenophaga strains [21] , [22] , none of which are alkaliphilic. Here we report the isolation and characterization of three different alkaliphilic strains (A1, B1 and H1) that are phylogenetically close to members of the genera Hydrogenophaga [21] and Malikia [23] from Barnes spring complex (BSC) in The Cedars [3] , [16] . We examine the three strains from geobiological, physiological, genomic, comparative genomic and environmental transcriptomic perspectives with a focus on understanding the ecophysiological properties; that is, how the microbes are environmentally distributed and how their metabolic activities potentially interact with the geochemistries of their environments. The isolated strains appear to be highly adapted to the long-lasting, very harsh geochemical conditions present in serpentinite-hosted terrestrial ecosystems. Isolation of strains A1, B1 and H1 Strains A1 and B1 were isolated from Barnes Spring 1 (BS1) while strain H1 was isolated from BS5 ( Supplementary Fig. 1 ), which are in the BSC, about 50 cm apart [3] . Both springs are fed mainly by the discharge of highly alkaline shallow groundwater [3] . 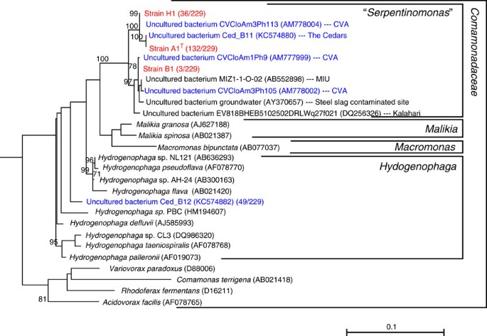Figure 1: Phylogenetic relationships among Betaproteobacterial 16S rRNA genes. Tree topologies are supported by bootstrap values for 100 replicates. Red font denotes strains isolated from Barnes spring complex in The Cedars and blue font denotes phylotypes recovered from the continental serpentinization sites including The Cedars. CVA: Cabeço de Vide, MIU: Mizunami Underground Research Laboratory, Kalahari: Kalahari shield. The water chemistries of the two springs are similar in terms of the pH (~\n 11.5), and ion and gas compositions ( Supplementary Table 1 ). DOC and total inorganic carbon in the water in BS5 pool were 20 μM and 70 μM, respectively, while bicarbonate ion levels (HCO 3 − ) were below the limit of detection (<2 μM) ( Supplementary Table 1 ) [3] . After initial enrichment on glass slides immersed in a mineral medium with hydrogen and acetate, pure colonies were isolated on Cedars Standard Media 1 (CSM1) plates. Single creamy/opaque colonies formed over a period of 2 weeks cultivation at 16 °C under gas mixture of 2.6% O 2 , 50% H 2, 9.8% N 2 and 37.6% Ar. The phylogenetic tree based on 16S rRNA gene sequences indicated that the three isolated strains were closely related to each other (>97.7% 16S rRNA gene identity) and clustered in family Comamonadaceae, order Burkholderiales , class Betaproteobacteria ( Fig. 1 ). 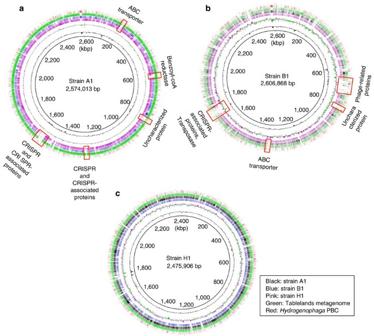Figure 2: Circular genome diagrams of the three isolated strains. Genomes for strain A1 (a), B1 (b) and H1 (c) are shown. The inner scales designate the coordinates (in kbp). The first (inner-most) circles show the GC contents and the second circles show the GC-skew. The third and fourth circles show the blastn analysis against the strain A1 (black), strain B1 (blue) and strain H1 (pink). The fifth and sixth circle show the blastn analysis against the metagenome of Tablelands35and the draft genome ofHydrogenophagasp. strain PBC22. The lower and upper identity threshold in the blastn analysis is >85 or >95, respectively. The locations of some genes of interest are indicated. The closest three genera are Hydrogenophaga [21] , Malikia [23] and Macromonas [24] , and the 16S rRNA gene similarities are summarized in Supplementary Table 2 . Figure 1: Phylogenetic relationships among Betaproteobacterial 16S rRNA genes. Tree topologies are supported by bootstrap values for 100 replicates. Red font denotes strains isolated from Barnes spring complex in The Cedars and blue font denotes phylotypes recovered from the continental serpentinization sites including The Cedars. CVA: Cabeço de Vide, MIU: Mizunami Underground Research Laboratory, Kalahari: Kalahari shield. Full size image Global distribution of related strains In total 464 environmental 16S rRNA clones were recovered from BS5 in the three separate field samplings between 2009 and 2011, and 49% of the clones were affiliated to the class Betaproteobacteria , which is the numerically dominant class of the microbial community in BS5 (ref. 16 ), although it should be kept in mind that this method is a semi-quantitative strategy for the community composition assessment. Detailed analyses revealed that 132, 36 and 3 of 292 clones for 16S rRNA gene were identical to those of the strains A1, H1 and B1, respectively; thus, the strain A1 and its close relatives (with 100% of 16S rRNA gene similarity) are the most dominant organism(s) and constitute ~\n28% of the bacterial community in BS5 ( Fig. 1 ). Further global distribution of phylotypes associated with strains A1, B1 and H1 was also examined and summarized in Table 1 . Strains A1, B1 or H1 related microbes (>99% identity in 16S rRNA gene sequences) were detected as one of the dominant phylotypes in most of the studied terrestrial serpentinizing environments including the Cabeço de Vide aquifer (CVA) in Portugal [17] , a Tablelands spring in Canada [18] and Outokumpu borehole water in Finland [20] ( Table 1 ). Further analyses revealed that phylotypes related to the isolated strains are abundant not only in actively serpentinizing terrestrial ecosystems, but also in man-made extremely alkaline industrial waste including hyperalkaline sediments surrounding a legacy lime (calcium oxide) working site in Buxton, United Kingdom [25] and microcosm experiments of groundwater from the Lake Calumet area of Chicago where the historic dumping of steel slag has filled in a wetland area [26] ( Fig. 1 , Table 1 , Supplementary Table 1 ). Microbes associated with strains A1, B1 or H1 were also detected in two slightly alkaline deep groundwaters where serpentinization is not suggested ( Supplementary Table 1 ): an ultra-deep granite groundwater in Mizunami [27] , Japan and borehole water from the 2.0 Ga Bushveld complex at the Evander mine in the Kalahari Shield, South Africa [28] ( Fig. 1 , Table 1 ). Table 1 Global distributions of strains A1, B1 or H1 associated phylotypes. Full size table In contrast, phylotypes associated with strains A1, B1 or H1 were not detected at two continental serpentinizing sites, the Leka ophiolite in Norway [19] and the Grotto pool spring 1 (GPS1) in The Cedars, California [16] , nor were they detected in any oceanic serpentinizing sites [29] , [30] , [31] . The geochemistry of the groundwaters from both the Leka ophiolite and GPS1 suggest that they are probably influenced by a marine component despite the fact that they are on land [3] , [32] ( Supplementary Table 1 ) for example, the alkaline water discharging from the GPS1 probably contacted the buried marine sediment below The Cedars peridotite. Thus, it appears that these strains are not tolerant of one or more components of the marine system. Overall, the common geochemical features of the sites where the strains A1, B1 and H1 related microbes were detected are alkaline conditions (pH 8.2–13), relatively high concentrations of calcium (0.5 mM–66 mM) and a relatively high ratio of Ca 2+ /Na + (>0.25) ( Supplementary Table 1 ). General physiological description of the strains Phase contrast observations revealed that the three isolated strains are motile rods that accumulate polyhydroxybutyrate (PHB) while growing in the presence of acetate ( Table 2 , Supplementary Fig. 2A–C ) [33] . The strains were unable to grow without the addition of vitamins and very little growth was observed when the cultures were shaken. Also, no growth was observed without the presence of CaCO 3 . Optimum growth for all the three strains was observed at 26–30 °C and at pH 11 when they were grown in liquid media ( Table 2 ). The optimum pH is the highest value for the any prokaryotes reported so far. The pH range for the growth varied slightly between the three strains. While the 4-[cyclohexylamino]-1-butansulphonic acid (CABS)-buffer ensured a stable pH during growth over a large range of pH values, it dropped to 11.5 when the initial pH value of the media was over 12 due to the out of the range buffer action [34] . Since the alkalinity of the medium at pH 12 represents 10 mM hydroxide, the initial pH is stable and the upper limit of growth can be derived from the initiation of growth at the given pH. Table 2 Summary of physiological characteristics of strains A1, B1 and H1. Full size table For all three strains, as growth progressed, the crystalline CaCO 3 precipitates were transformed into amorphous structures ( Supplementary Fig. 3 ). Observations by confocal laser scanning microscopy revealed that the strains formed aggregates on the CaCO 3 precipitates and that the size of the microbe CaCO 3 complex became larger as they grew ( Supplementary Fig. 4 ). All three strains grew with a broad range of oxygen (2.5–20%) in the headspace, and the growth was inhibited by NaCl at concentrations above 0.5 g l −1 . 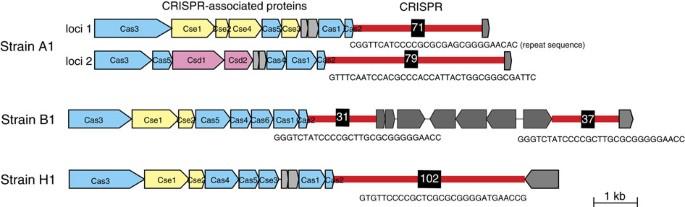Figure 3: Comparisons of predicted CRISPR and CRISPR-associated proteins in strains A1, B1 and H1. Coloured boxes represent Cas (blue), Cse (yellow), Csd (pink) and unrelated proteins (gray). Red bars show the consensus repeats and spacer regions and numbers in black box indicate the numbers of repeats. Utilization of substrates and electron acceptors The three strains grew heterotrophically with a wide range of carbon substrates including various fatty acids and sugars ( Table 2 , Supplementary Table 3 ). In addition, they all grew autotrophically with hydrogen (electron donor), CaCO 3 precipitate (carbon source) and oxygen (electron acceptor) ( Table 2 , Supplementary Fig. 5 ). Thin sectioning transmission electron microscope (TEM) observation of strain A1 revealed the presence of carboxysome-like structures after 5 days of autotrophic growth ( Supplementary Fig. 6A ), and abundant PHB accumulations were observed in mixotrophically grown cells with hydrogen, oxygen, CaCO 3 and acetate ( Supplementary Fig. 6B ). Some differences among the three strains were observed with regard to substrate or electron acceptor utilization, as judged by consumption of substrate(s) or electron acceptor(s), byproduct production and/or cell growth. Strains B1 and H1 (but not A1) grew well via sugar fermentation ( Table 2 ). Strain A1 utilized cyclohexane well as its substrate, which likely originated from the deep groundwater source in The Cedars spring water [3] , while strain B1 and H1 showed a limited or no growth with cyclohexane, respectively. With regard to electron acceptor utilization, all strains utilized oxygen as an electron acceptor, while only strain A1 utilized thiosulphate with sulphide as one of its products and strains B1 and H1 utilized nitrate ( Table 2 ). Strain H1 also used nitrite as an acceptor, but the product was not measured. Genomic features of strains A1, B1 and H1 Draft genome sequences of the three strains were determined, and gap-closing efforts were made for strains A1 and B1 ( Table 3 , Supplementary Fig. 7 ). The genomes were similar with regard to: (1) size, all were approximately 2.5 Mb, which is significantly smaller than those of closely related sequenced strains within class Betaproteobacteria ; (2) G+C content; and (3) rRNA gene-copy number. However, strains B1 and H1 possess a plasmid (16 kbp), which was not present in strain A1. The plasmid sequences from strains B1 and H1 are highly conserved with 99.85% identity, but contain no recognizable metabolism-related genes. Table 3 Genomic features of strains A1, B1 and H1, and most closely related strains. Full size table Genome-wide comparisons of strains A1, B1 and H1 ( Fig. 2 ) showed that the three strains, especially strains A1 and H1, are highly similar in their genomes; however, all three strains were significantly different from Hydrogenophaga sp. strain PBC, the only strain within this genus that has had its genome sequence published ( Fig. 2 , Table 3 ) [22] . A metagenomic sequence of the microbial community in spring WHC2B at Tablelands, which was published by Brazelton et al. [35] , showed high similarity with strains A1 and H1 ( Fig. 2a,c ). Further blastn analyses with higher threshold (lower threshold >90% and upper threshold >95%) revealed that the sequences from Tablelands community contain highly conserved strain A1-like genomes in the metagenome ( Supplementary Fig. 8A ). Figure 2: Circular genome diagrams of the three isolated strains. Genomes for strain A1 ( a ), B1 ( b ) and H1 ( c ) are shown. The inner scales designate the coordinates (in kbp). The first (inner-most) circles show the GC contents and the second circles show the GC-skew. The third and fourth circles show the blastn analysis against the strain A1 (black), strain B1 (blue) and strain H1 (pink). The fifth and sixth circle show the blastn analysis against the metagenome of Tablelands [35] and the draft genome of Hydrogenophaga sp. strain PBC [22] . The lower and upper identity threshold in the blastn analysis is >85 or >95, respectively. The locations of some genes of interest are indicated. Full size image In all, 48.5% of raw reads from the Tablelands metagenome were assigned to the order Burkholderiales where our isolated strains belong [35] and 9 out of the 10 longest contigs assembled from the Tablelands metagenome showed high similarity with the genome of strain A1 ( Supplementary Fig. 9 ), implying that A1-like microbe(s) are numerically dominant in the Tablelands as well. Detailed comparisons between strain A1 genome and the nine long contigs from Tablelands metagenome indicated that the genome sequences are highly similar except for large indel sequences and/or gene translocations that were observed between the two ( Supplementary Fig. 9 ). Some gene clusters of strains A1, B1 and H1 are unique to the genome of each strain, including gene clusters encoding Clustered Regularly Interspaced Short Palindromic Repeats (CRISPRs) and CRISPR-associated proteins ( Fig. 3 ), which are known to be responsible for prokaryotic immunity to phage infection [36] . Detailed comparisons of the CRISPR sequences revealed no similarity between the strains with regards to the numbers of repeats, consensus repeat and spacer sequences. The results may imply a different history of phage interaction for the isolated strains in their respective environments, regardless of the physiological and genomic similarity of the three. While low similarities were observed in CRISPR region between strain A1 and the Tablelands metagenome, several CRISPR-associated proteins showed some similarities. However, all CRISPR-associated proteins from Tablelands metagenome were on short contigs, suggesting that the sequence assemblies of the Tablelands metagenome may be limited in this region due to the repeat sequences contained in CRISPR [35] . Figure 3: Comparisons of predicted CRISPR and CRISPR-associated proteins in strains A1, B1 and H1. Coloured boxes represent Cas (blue), Cse (yellow), Csd (pink) and unrelated proteins (gray). Red bars show the consensus repeats and spacer regions and numbers in black box indicate the numbers of repeats. Full size image Metabolic pathways possibly required for inhabiting The Cedars springs Presence and absence of the gene sets that are assumed to be important for inhabiting this environment within the genomes of three strains were selected and summarized in Fig. 4 . 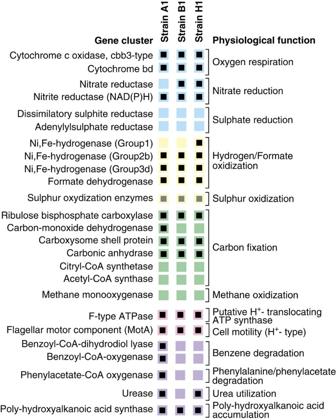Figure 4: The presence of selected biosynthetic/catabolic genes or gene clusters in the sequenced strains. Black squares represent the presence of a gene or entire gene cluster within a genome. Grey squares represent partial presence of the gene cluster. Coloured boxes represent genes or gene clusters related to respiration (blue), electron donation (yellow), carbon fixation (green), energy production (pink) and other metabolisms (purple). Figure 4: The presence of selected biosynthetic/catabolic genes or gene clusters in the sequenced strains. Black squares represent the presence of a gene or entire gene cluster within a genome. Grey squares represent partial presence of the gene cluster. Coloured boxes represent genes or gene clusters related to respiration (blue), electron donation (yellow), carbon fixation (green), energy production (pink) and other metabolisms (purple). Full size image With regard to electron acceptor utilization, all strains have the entire gene complements required for oxygen respiration. In agreement with the physiological analyses, strains B1 and H1 have a nitrate reductase gene cluster, while strain A1 lacks it. The genes encoding dissimilatory thiosulphate reductase such as phs genes were not detected in any of the three [37] , although strain A1 was able to reduce thiosulphate and produced sulphide in the physiological analyses. Well-known electron donors utilized for microbial autotrophic growth are hydrogen and reduced forms of sulphur (sulphide, S 0 , thiosulphate). Hydrogenase is a key enzyme for autotrophic growth with hydrogen. Strains A1 and B1 have two gene clusters encoding different [NiFe]-hydrogenases while strain H1 has three. Functional clustering of the resulting [NiFe]-hydrogenase based on the report from Vignais et al. [38] revealed that all three strains have the hydrogenases clustered into Group 2b and 3d, and only strain H1 has an additional hydrogenase clustered in Group 1 ( Fig. 5 ). The hydrogenases in Group 1 are known as membrane-bound, respiratory uptake H 2 ases capable of supporting growth with H 2 as an energy source [38] . However, despite the fact that all three can grow autotrophically, Group1 hydrogenase was detected only in the genome of strain H1. Thus, apparently this type of uptake hydrogenases is not a necessary complement for growth on hydrogen in this taxon. Hydrogenases clustered in Group 2b are known for the involvement in H 2 sensing but they are not directly involved in energy production [38] . Meanwhile, hydrogenases clustered in Group 3d are cytoplasmic enzymes and share extensive similarity to the peripheral part of bacterial respiratory Complex 1. The Group 3d hydrogenase is considered to be able to link directly to hydrogen in the cytosol and reduce NAD + to NADH for supplying the NADH to the carbon fixation [38] , [39] . In principal, the NADH could also be used as energy source; therefore, the hydrogenase in Group 3d may be highly important in autotrophic growth of the isolated strains. 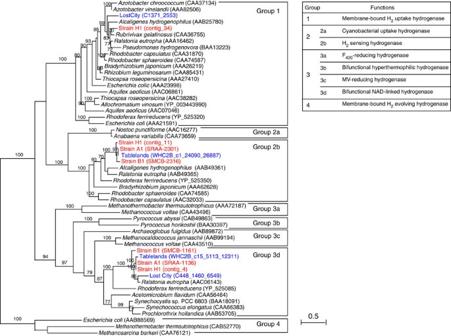Figure 5: Phylogenetic diversity of putative [NiFe]-hydrogenases from strains A1, B1 and H1, and from Tablelands metagenomes. Red font denotes the putative hydrogenases from strains A1, B1 and H1 and blue font denotes the putative hydrogenases recovered from the Tablelands spring fluid. Group numbers are consistent with the phylogeny reported by Vignaiset al.38Maximum-likelihood bootstrap support values >70 are shown. Figure 5: Phylogenetic diversity of putative [NiFe]-hydrogenases from strains A1, B1 and H1, and from Tablelands metagenomes. Red font denotes the putative hydrogenases from strains A1, B1 and H1 and blue font denotes the putative hydrogenases recovered from the Tablelands spring fluid. Group numbers are consistent with the phylogeny reported by Vignais et al. [38] Maximum-likelihood bootstrap support values >70 are shown. Full size image While partial gene clusters related to sulphur oxidation were detected (only sox YZ) in all three genomes ( Fig. 4 ), other putative sox genes were not seen. Although only strain A1 showed the thiosulphate oxidation accompanied with autotrophic growth, potential genes related to thiosulphate oxidation were not detected in the strain ( Table 2 ). With regard to inorganic carbon fixation, all three strains have most of the genes and gene clusters encoding enzymes of the Calvin-Benson cycle [40] while the key genes that are essential for the reverse TCA cycle (Citryl-CoA synthetase) [41] , [42] and reductive acetyl-CoA pathway (Acetyl-CoA synthase) [43] are not present, suggesting that carbon dioxide fixation is occurring via the Calvin-Benson cycle ( Fig. 4 ). In addition, the genes encoding carboxysome shell proteins and a carbonic anhydrase are present in all three genomes, which also support the usage of the Calvin-Benson cycle for carbon fixation [44] . Only strain A1 has putative cox genes (form I) that encode a carbon-monoxide (CO) dehydrogenase (CODH) [45] , [46] , which was also seen in the Tablelands metagenome. Similar cox genes were detected in Hydrogenophaga pseudoflava that utilizes CO as an energy source [47] , suggesting that strain A1 also may utilize CO as energy source. No physiological tests of growth on CO were attempted. The genes required for carbon fixation were located in a particular region in the genomes or contigs ( Supplementary Fig. 10 ). The sequence comparisons of this region in the genomes between strains A1 and B1 as well as contigs from the strain H1 and the metagenome of Tablelands [35] indicate that the region is highly conserved. In concert with the genomic similarities between strain A1 and the Tablelands metagenomic contig noted above, the carbon fixation region also showed the highest similarities among the four compared sequences for these two. The region including CODH was also presumably an indel sequence, although the contigs from strain H1 and Tablelands were not long enough for a detailed comparison. With regard to aromatic organic carbon metabolism, genes encoding benzene degradation and phenylalanine/phenyl-acetate degradation were also detected but only in strain A1. As aromatic compounds and cyclohexane were detected in BS5 water [3] , the feature also may contribute to support the life there. Although some alkaliphilic microbes are known to utilize sodium ions instead of protons for energy metabolism in alkaline settings [48] , [49] , the comparisons of the amino-acid sequences of F-type ATPase subunit c indicate that ATPases in the three strains are likely H + -translocating ATP synthase as is commonly observed in aerobic alkaliphilic microbes ( Supplementary Fig. 11 ) [50] . However, in contrast to the well-investigated highly alkaliphilic strain Bacillus pseudofirmus OF4 (ref. 49 ), the presence of motA [51] , the gene encoding the component of the H + -driven bacterial flagellar motor protein, suggests that the flagella-mediated motility of these isolates is also likely driven by a proton gradient: no Na + -driven motor proteins were detected ( Fig. 4 ) [52] . Therefore, regardless of having the highest optimum pH, the strains presumably utilize a proton motive force (PMF) for energy production. Expression of autotrophic growth-related genes in strain A1 Autotrophic growth with hydrogen as electron donor and calcium carbonate as carbon source is probably an effective metabolism in an environment with low concentrations of organic carbon and abundant hydrogen and calcite. To confirm the occurrence of autotrophic growth in The Cedars site, gene expression analyses, targeted to the genes presumably required for autotrophic growth, were conducted with the DNA and RNA recovered from the microbial community in BS5 spring water ( Fig. 6a ), and also RNAs prepared from strain A1 culture grown autotrophically or mixotrophically ( Fig. 6b ). Strain A1 was not able to grow without CaCO 3 and also the growth was significantly inhibited in the absence of hydrogen. Therefore, RNAs from strain A1 grown heterotrophically could not be prepared. The primers were designed for detecting the genes from strain A1 specifically, but given the high similarities among the three strains, some of the primers may detect genes from two or three of the strains as well as other related substrains for the in situ gene expression analysis. Thus, the gene expression levels were evaluated by the cDNA/DNA ratio for the environmental sample, as shown in Fig. 6 . Using this approach, all genes targeted in this study were confirmed to be present in the environmental DNAs and expressed to some extent. 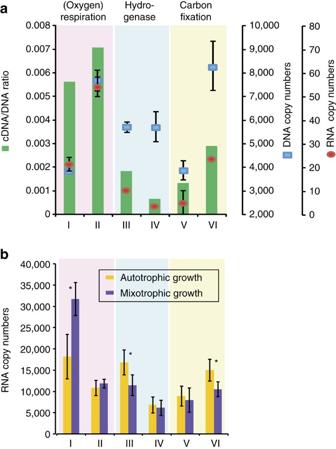Figure 6: Gene expression analyses of autotrophic growth-related genes from strain A1. (a)In situgene expression analysis. Blue squares indicate the copy numbers of each gene in 2.5 ng of DNA recovered from microbial communities in BS5 spring fluid. Red circles indicate the copy numbers of each gene’s transcripts in the synthesized cDNA corresponding to 25 pg of RNA recovered from the microbial community in BS5 spring fluid. Green bars indicates cDNA/DNA ratio of each gene. The targeted genes shown as I-VI encode the following proteins: I; Cbb3-type cytochrome oxidase, subunit 1 (SRAA-0853), II; NADH dehydrogenase subunit D (SRAA-0747), III; [NiFe]-hydrogenase in Group 3d (HoxH) (SRAA-1136), IV; [NiFe]-hydrogenase in Group 2 (SRAA-2301), V; Aerobic-type carbon monoxide dehydrogenase, large subunit CoxL/CutL homologs (SRAA-2294) and VI; Ribulose 1,5-bisphosphate carboxylase, large subunit (Rbc L) (SRAA-2317). Bars indicate s.d.(±s.d.,n=3). (b)In vitrogene expression analysis. Yellow and purple bars indicate the copy numbers of each gene’s transcripts in the RNAs (cDNA) recovered from strain A1 grown autotrophically (yellow) and heterotrophically (purple). Differences between values in two conditions followed by asterisks are significant(P<0.01, Student’st-test) (n=3). Figure 6: Gene expression analyses of autotrophic growth-related genes from strain A1. ( a ) In situ gene expression analysis. Blue squares indicate the copy numbers of each gene in 2.5 ng of DNA recovered from microbial communities in BS5 spring fluid. Red circles indicate the copy numbers of each gene’s transcripts in the synthesized cDNA corresponding to 25 pg of RNA recovered from the microbial community in BS5 spring fluid. Green bars indicates cDNA/DNA ratio of each gene. The targeted genes shown as I-VI encode the following proteins: I; Cbb3-type cytochrome oxidase, subunit 1 (SRAA-0853), II; NADH dehydrogenase subunit D (SRAA-0747), III; [NiFe]-hydrogenase in Group 3d (HoxH) (SRAA-1136), IV; [NiFe]-hydrogenase in Group 2 (SRAA-2301), V; Aerobic-type carbon monoxide dehydrogenase, large subunit CoxL/CutL homologs (SRAA-2294) and VI; Ribulose 1,5-bisphosphate carboxylase, large subunit (Rbc L) (SRAA-2317). Bars indicate s.d. (±s.d., n =3). ( b ) In vitro gene expression analysis. Yellow and purple bars indicate the copy numbers of each gene’s transcripts in the RNAs (cDNA) recovered from strain A1 grown autotrophically (yellow) and heterotrophically (purple). Differences between values in two conditions followed by asterisks are significant (P <0.01, Student’s t -test) ( n =3). Full size image The gene encoding Cbb3-type cytochrome oxidase, which is responsible for oxygen respiration, is highly expressed and the gene encoding NADH dehydrogenase, which is a key enzyme to generate proton motive force, is also significantly expressed ( Fig. 6a ). Although dissolved oxygen was below detection level in the BS5 pool, the E h at the depth of 1, 3, 10, 20 and 40 cm below the surface was −40, −93, −182, −251 and −550 mV, respectively [16] . Thus, the E h gradient suggests that not only is atmospheric O 2 dissolving into BS5 pool, but it is also probably being consumed biotically [16] . These results suggest that strain A1 uses oxygen as the electron acceptor and generates energy in the field. These genes were also expressed in the in vitro examination, while the gene encoding Cbb3-type cytochrome oxidase was expressed significantly higher under the mixotrophic growth condition ( Fig. 6b ). The gene encoding the hydrogenase clustered in Group 3d is highly expressed, while that in Group 2 is poorly expressed in the environment ( Fig. 6a ). The in vitro study indicates that the Group 3d hydrogenase is correlated with the autotrophic growth ( Fig. 6b ) as predicted by the functional clustering [38] , [39] . Thus, strain A1 presumably utilizes environmental hydrogen by using the Group 3d hydrogenase. With regard to the genes related to inorganic carbon fixation, the gene for large subunit of Rubisco ( rbcL ) was highly expressed in the environment while the gene encoding CODH ( coxL ) was poorly expressed ( Fig. 6a ). The in vitro study indicates that the expression of the rbcL was enhanced significantly during the autotrophic growth while the expression of the coxL was similar during autotrophic or mixotrophic growth. ( Fig. 6b ). Thus, the Calvin-Benson cycle, which has a Rubisco in the pathway, appears to be method of carbon fixation in the environment. Proposal for a new genus The three isolated strains from The Cedars are distinct from the genera Hydrogenophaga , Malikia and Macromonas as indicated in the phylogenetic tree ( Fig. 1 ) and 16S rRNA gene similarity ( Supplementary Table 2 ). In addition, many physiological properties also distinguish them from the previously known genera. Therefore, we propose strains A1, B1 and H1 as a new genus Serpentinomonas and strain A1 as the type strain of this genus. Generally, in species-level taxonomic comparisons, DNA-DNA hybridization is known as the most confident way for describing the genetic distance of multiple strains [53] . On the basis of the principal of DNA-DNA hybridization strategy, in silico DNA-DNA hybridization was employed for determining the species level taxonomy of these three ( Supplementary Fig. 12 ). When 80% of similarity cutoff and 95% of length cutoff were applied for the mapping, strains A1 and H1 shared more than 70% of genome similarity; however, strain B1 shared only around 50% with the other two strains, suggesting that strains A1 and H1 can be considered as one species while strain B1 is different. Thus, we propose three strains isolated from The Cedars springs as a new candidate genus and species Serpentinomonas raichei strain A1 T and H1, and Serpentinomonas mccroryi strain B1, respectively. A formal description of the new taxa will be reported elsewhere. The Serpentinomonas strains described here are obligatory alkaliphilic and facultative hydrogen-utilizing bacteria. Closely related strains were numerically dominant microbes in various terrestrial active serpentinizing sites around the globe ( Table 1 ). Thus, it would appear that these strains are very relevant to understanding the interactions between the geochemistry of terrestrial serpentinization sites and the microbes that inhabit them. Abiotically released Ca 2+ in a highly alkaline environment reacts rapidly with DIC to form insoluble calcium carbonate ( Supplementary Fig. 1 ) [3] , [9] . Under such limiting conditions of DIC, Serpentinomonas strains utilize CaCO 3 for carbon fixation, coupled with hydrogen oxidation at high pH. Thus, the Ca 2+ released in the alkaline water appears to be a great carbon-trapping mechanism for the Serpentinomonas microbes. To our knowledge, no microbe capable of fixing carbon at that high pH using calcium carbonate as the source of inorganic carbon has been reported. The possible explanation of the phenomenon for the utilization of CaCO 3 at pH 11 is that the strains aggregate on CaCO 3 and may decrease the pH in the microenvironment surrounding them by generating a proton gradient, ( Supplementary Fig. 4 ), thus converting the soluble carbonate released from the calcite to produce bicarbonate for immediate carbon uptake. An alternative explanation is that the Serpentinomonas strains may have extremely high affinity bicarbonate transporter(s), and these strains closely attach to CaCO 3 and may locally increase the solubility of calcium carbonate. In either case, the fixed carbon from CaCO 3 by the strains could affect to the other community members’ metabolisms by providing the organic carbons. In addition to the autotrophic growth strategy, Serpentinomonas strains have diverse metabolic abilities in terms of organic carbon compound and electron acceptor utilization ( Table 2 , Supplementary Table 3 ). The ‘edge of life’ conditions with regard to highly limiting electron acceptors and carbon sources during evolution may have stimulated an opportunistic life style with regard to available substrates and thus may have facilitated the acquisition of the diverse metabolic capabilities. In addition, varying CRISPR immune components in each strain indicate that the histories of virus (phage) infection are different [36] ( Fig. 3 ). Because of the harsh environment, microbial competitors of these strains are probably not abundant, and eukaryotic predators are virtually absent [16] , but the virus infection may be an important component for the genetic exchange between microbes in The Cedars springs. Given their small genome size in comparison with taxonomically similar microbes living in less challenging environments, it appears that many excess genes have been lost via genome streamlining [54] , [55] , [56] . An alternative hypothesis is that these microbes are the ‘precursors’ of other ‘more modern’ microbes, which have achieved their genomes by accretion of new genes [56] . Although the organisms are clustered into the family Comamonadaceae, the latter hypothesis might be more compatible with the observation that genomically close strains are seen in globally separated ecosystems and also highly related strains are seen in present day serpentinization of Precambrian shield and other younger serpentinite ecosystems. In such harsh environments, with few predators, and consistently harsh and relatively stable conditions, there may be little advantage to change and/or diverge. Environmental and in vitro gene expression profiles indicate the occurrence of autotrophic growth with hydrogen, oxygen and carbon dioxide in The Cedars spring. On the basis of the genomic and transcriptomic analyses in this study, we assumed that Serpentinomonas strains utilize cytoplasmic hydrogenase (Group 3d), which can link hydrogen directly and reduce NAD + to NADH, for the hydrogen oxidation accompanied with the energy production. Since this enzyme normally links to Complex I of the respiratory chain, this route would potentially yield more energy than the (periplasmic) Group I hydrogenase, which links to the Q-pool of the respiratory chain [57] . In addition, in the highly alkaline and hydrogen-rich environment, hydrogen oxidation in the cytosol may be more effective with regard to the energy production. The physiological functions of the different hydrogenases must be further analysed since the hydrogenases obviously are very important in creating a proton motive force and cytoplasm homeostasis at this high pH. One of the mysteries of the Serpentinomonas strains relates to their energy metabolism and homeostasis. The study of an alkaliphilic gram-positive bacteria, B. pseudofirmus OF4, proved that the strain developed several strategies to adapt pH>10 including alkaliphile-specific features of the ATP synthase (for example, changes at the c-ring’s ion binding site as well as its size and stoichiometry) [58] and also delocalized gradients near the membrane surface and proton transfers to ATP synthases via membrane-associated microcircuits between the proton pumping complexes and synthases [49] . Since the Serpentinomonas strains are gram-negative bacteria, grow well only above pH 10.5 and the important protein motif in c-ring of ATPase (AxAxAxA) in strain OF4 (ref. 58 ) was not detected in that of Serpentinomonas strains, the Serpentinomonas strains may have a different strategy of adaptation to the calcium-rich and sodium-poor ultrabasic environment. In conclusion, the ‘edges of life’ conditions found at continental serpentinizing environments appear to have selected for quite similar Serpentinomonas strains. In this study, we revealed various aspects of Serpentinomonas strains’ characteristics, especially focused on the ecophysiological perspective. Through this study, further questions and hypotheses have been raised concerning the microbial evolution and energy metabolism of Serpentinomonas strains. Answering those must provide further new insights into microbial life on modern or perhaps early Earth. Sampling sites and sample collections Water samples for microbial isolations were collected from BS1 and BS5 (BSC: elevation 282 m, N: 38°37.282′, W: 123°7.987′) within The Cedars [3] and used for various liquid enrichments in basal media supplemented with or without organic substrates (see ‘Medium composition’). Since no visible turbidity developed, pre-autoclaved glass slides or glass beads (0.11 mm diameter ballotini beads) were incubated in situ in the BS1 pool, just above the entry of the spring in the pool at E H of around −250 to 350 mV in July 2005. After 1–2 weeks, microscopic inspection showed profuse growth on the slides or beads. The slides and beads were used for enrichments in the laboratory (see below). BS5 water was collected in October 2010 and directly used for enrichments. Cell samples for DNA and RNA analyses were pumped and collected from the water in BS5 pool with Tygon Chemical Tubing (Masterflex) equipped with PFA In-Line filter holders (Advantec) in 2011 (ref. 16 ). The 0.22-μm in-line filters (Millipore) were used for microbial cell collection. The water flow rate was ~\n150 ml min −1 and the filter was exchanged every 30 min. The filtered cells were frozen immediately with dry ice at the sampling site and kept at dry ice temperature during the transportation. Final water volume filtered for the DNA and RNA extraction was ~\n150 l. Bacterial isolation Water samples, preincubated slides or beads were used as inoculum for further liquid enrichments in the laboratory in basal (minerals+vitamins) medium (pH 9.5–11.5) supplemented with 30% (v/v) prefiltered BS1 or BS5 water and incubated at 16–18 °C with and without various organic substrates in an atmosphere of H 2 (0.25–0.50 atm), CH 4 (0.0–0.25 atm), O 2 (0.05 atm) and N 2 or Ar (0.45 atm), with immersed ballotini beads or a glass slide as support. After 1–2 weeks, the enrichments in the liquid or on the glass surface were streaked on basal agar media with 2 mM acetate for the development of colonies in the same gas mixture at 16–18 °C. Slightly different creamy/opaque colonies obtained from pool BS1 were restreaked at least five times to obtain pure cultures and labelled strain A1 and B1. After suspension, the strains were stored in glycerol (20% v/v) at −80 °C, in 2005. Strains A1 and B1 were revived from the stored colonies in 2010 for physiological tests and further cultivated in an atmosphere of O 2 /H 2 /N 2 /Ar 2.6:50:9.8:37.6 by volume (1 atm) at 16 °C. If H 2 was not desired in the medium, it was replaced by N 2 or Ar. BS5 pool water collected in 2010 was directly used for enrichments in the laboratory at 16–18 °C on basal medium supplemented with 30% prefiltered BS5 water under the same gas atmosphere. The liquid medium, supplemented with 4 mM acetate, contained a glass slide to promote visible attached growth. From this enrichment strain H1 was isolated in pure culture, as described for strains A1 and B1, on basal agar medium with acetate under O 2 /H 2 /N 2 /Ar 2.6:50:9.8:37.6 by volume (1 atm) Pure cultures were grown at 16 °C in liquid basal media with acetate, concentrated by (aseptic) centrifugation and then stored in glycerol (20% v/v) at −80 °C. Medium composition Media consisted of ‘basal’ Cedars Standard Medium 1 (CSM1) supplemented with a large range of organic substrates at 0.5–4 mM concentrations adjusted to various pH. Acetate was used at 2–4 mM. The CSM1 contained 0.05 mM Na 2 SO 4 , 0.378 mM NH 4 Cl, 0.05 mM MgCl 2 , 0.06–0.115 mM K 2 HPO 4 (matching the 2 or 4 mM acetate concentration used), 2.00 mM CaCO 3 (as suspension), 10 mM CABS or Na 2 CO 3 /NaHCO 3 , 10 ml l −1 of ATCC Trace Mineral Supplement and 10 ml l −1 of ATCC Vitamin Solution (or self-prepared basic vitamin solution, with concentrations identical to those in ATCC Vitamin Solution but without KH 2 PO 4 ). The pH of the CSM1 was adjusted by using NaOH. For optimum growth, the pH was adjusted to 10.5–11.2 and the temperature was 16–18 °C. Since the cell growth could not be monitored by the optical density due to the low cell density as well as the precipitate of calcium carbonate, the cells were stained with SYBR Green I and collected on black filters and monitored under fluorescent microscopy, or monitored by directly placing the glass slides under the phase-contrast microscope. Pure colonies were isolated on CSM1 plates supplemented with 2–4 mM acetate, with 2% prewashed Noble (Difco) or Korean (Daishin) agar (Brunschwig Chemie, Amsterdam, NL). Small (0.2–1 mm) creamy/opaque colonies formed over a period of 2 weeks cultivation at 16 °C under a gas mixture of O 2 /H 2 /N 2 /Ar 2.6:50:9.8:37.6 by volume (1 atm). Once the temperature optimum and pH optimum was determined, cultures were routinely grown at 28 °C and pH 10.8–11.2. 3-(Cyclohexylamino)-1-propanesulphonic acid (CAPS) (Sigma) was used instead of CABS in a gas mixture of O 2 /H 2 /N 2 or Ar 2.6:50:47.4 by volume (1 atm). Although initial enrichments and isolations were performed in the condition described above, the cultivation condition was optimized for the further physiological examinations. The basal liquid media for the physiological analysis (Cedars Standard Media 2 (CSM2)) was composed with 0.1 mM Na 2 SO 4 , 0.755 mM NH 4 Cl, 0.1 mM MgCl 2 , 0.23 mM K 2 HPO 4 , 20.0 mM CaCO 3 (as suspension), 15 mM CAPS and self-prepared Trace Mineral and Vitamin Solution [59] . The portion for the liquid and gas phase is approximately 35:65. The gas composition is H 2 /N 2 /Air 35:35:30, the temperature for the cultivations is at 30 °C and 4 mM of sodium acetate was added unless otherwise noted. Physiological characterization The optimum and range of pH, temperature and sodium chloride concentrations for the growth were evaluated by the increase in cell numbers and consumption of acetate. For electron donor or carbon source examinations, the 4 mM of substrates listed in Supplementary Table 3 was added instead of 4 mM of sodium acetate. N 2 /Air=7:3 was used as the gas phase for the electron donor examination while the gas phase contained H 2 (see above) was used for the carbon source examination. The growth was confirmed by the increase in cell numbers compared with those of the controls. In addition, the consumptions of acetate, propionate, butyrate, lactate hydrogen were confirmed. Pyruvate and formate were not accurately measured in our system due to the instability of compounds. The growth with glucose, glutamate, glycerol and cyclohexane was evaluated only from the increase in cell numbers. In the examinations of electron acceptor utilizations, N 2 /H 2 =5:5 (except for the oxygen utilization) was used for the gas composition and the electron acceptor availability was evaluated the increase of cell number and consumption of acetate. In addition, the reduction of the nitrate, sulphate, thiosulphate and iron was evaluated by nitrite, sulphide or iron (II) productions. Nitrite, sulphide and iron (II) were detected with Griess [60] , methylene blue [61] or ferrozine methods [62] , respectively. HPLC and gas chromatography Volatile fatty acid (VFA) (acetate, propionate, butyrate, lactate) concentrations in the media were measured using a HPLC machine equipped with a multiple wavelength detector (Agilent 1200 series) and a reverse phase C18 column [59] (Epic Polar, ES Industries or Synergi 4 μm Hydro-RP 80 Å, Phenomenex). The eluant was 50 mM phosphoric acid (pH 1.87) for Epic Polar and 0.5 mM sulphuric acid (pH 2.61) for Synergi 4 μm Hydro-RP 80 Å at a flow rate of 1.0 ml min −1 . Acetate, propionate, butyrate and lactate were identified and determined based on known standards (detection limit was>0.1 mM). Hydrogen gas concentration was measured by GC (CP-3800, Varian) using a Fused Silica Molsieve 5A column (CP7537, Varian). Hydrogen peaks and concentrations were identified with the comparison with the standard and the standard curve prepared with pure hydrogen. Microscopy For both confocal laser scanning microscopy (confocal microscopy) and TEM, bacterial cells were grown autotrophically with H 2 , O 2 and CaCO 3 or mixtrophically with H 2 , O 2 , acetate and CaCO 3 . Confocal microscopic observation was made for the bacterial cells grown for 3 days under the condition described above. The samples were collected by needle from the bottle with bacterial culture. The collected cells were stained with SYBR green I (Life Technologies) and observed directly under confocal microscopy. For TEM observation, bacterial cells grown for 5 days were harvested by centrifugation, fixed with 2.5% glutaraldehyde in 0.1 M sodium phosphate buffer (pH7.4) at 4 °C for 5 h and then postfixed with 2% osmium tetroxide for 90 min at 4 °C. The fixed cells were embedded in 1.5% agarose before dehydration with a graded ethanol series. The dehydrated specimens were embedded in Epon812 resin. Ultrathin sections of the samples were prepared with a Reichert-Nissei ultramicrotome (Ultracut-N), mounted on copper grids and stained with 1% uranyl acetate and 0.3% lead citrate. Images of sections were obtained by using a Hitachi model H-7600 transmission electron microscope operating at 80 kV. Sequencing and sequence assembling DNAs from Serpentinomonas strains for the genomic sequencing were extracted using the MObio PowerBiofilm DNA Isolation Kit (MObio). The prepared DNA was used for library construction for Illumina Hiseq. Paired-end libraries were prepared using Bioo Scientific NEXTflex Library Prep Reagents for Illumina kit and protocol, with Bioo Scientific NEXTflex PCR-Free Barcoded adapters. Cluster generation and sequencing were conducted by employing the 101-bp read length option. Paired-end sequencing approaches were conducted by Illumina’s standard protocol. Total reads generated from the sequencing were 3,857,324, 4,385,866 and 5,253,809 for strain A1, B1 or H1, respectively. The de novo assembly of genomic sequences was primary conducted using the Velvet assembler. The assembled contigs were compared with those from CLC assembly (Version 6.0.3) and the contig for each strain was finalized. The assembled stats are shown in Supplementary Table 4 . The contig gaps in strains A1 and B1 genomes were closed by PCR-based primer walking. As for strain H1, over 300 bp of contigs (93 contigs for the chromosome and 1 contig for the plasmid) were applied for the further genomic analyses. Environmental DNA and RNA extraction Several chemical and mechanical cell disrupting methods were examined for effectively extracting total nucleic acids from the microbial cells inhabiting in The Cedars highly alkaline fluid, and a modified MObio PowerBiofilm RNA Isolation Kit (MObio) was selected to achieve the highest yield of total nucleotide. The standard MObioRNA extraction method was followed with modifications described here. First, the frozen cells on the filter were directly added to the power beads containing Solution BFR1/β-mercaptoethanol. After inhibitor removal steps, we skipped the DNA removal process and moved to the washing step [63] . Extracted total nucleic acids were separated using the AllPrep DNA/RNA Mini Kit (Qiagen). RNA from strain A1 was also prepared using MObio PowerBiofilm RNA Isolation Kit according to the manufacturer’s instruction. Gene expression analyses cDNAs were synthesized from the prepared RNAs using SuperScript VILO cDNA Synthesis Kit (Life technologies). Twenty nanograms of total RNAs from the environmental cell samples and 10 ng of total RNAs prepared from the 250 ml of strain A1 culture ( n =2) were applied for the cDNA synthesis. The qPCR analysis was conducted using Fast SYBR Green Master Mix with the 7500 Fast Real-Time PCR System (ABI) ( n =3) and the single-amplicon production in each reaction was confirmed by the dissociation curve. All the procedures for the qPCR were conducted following the manufacturer’s instruction. The primer sequences targeting six analyzed genes are shown in Supplementary Table 5 . Gene and genome analyses The open-reading frame (ORF) predictions and annotations for the assembled genomes and contigs were conducted using Migap ( http://www.migap.org/index.php/en ) [64] . The 16S rRNA gene sequences were aligned with cmalign (v1.1rc1) from the Infernal package and trimmed with TrimAl (v1.2rev59) for the phylogenetic tree construction [16] . The hydrogenase protein sequences were aligned with Muscle [65] . The trees were created by using maximum-likelihood with RaxML, and the robustness of furcated branches was supported by bootstrap values (100 replicates) [66] A BLAST Ring image generator was employed for visualizing a prokaryote genome as a circular image with multiple prokaryote genome comparisons [67] . GenomeMatcher was used for the comparisons of contigs with the ‘compare sequence’ mode [68] . In silico DNA-DNA hybridization The raw reads from strains A1, B1 and H1 sequencing (average read length=101 bp) were mapped to each gap-closed or draft genome using CLC (Version 6.0.3). The cutoff parameters that we have attempted are 95 for the similarity cutoff while 70, 80 and 90 for the length cutoff. Accession codes: The genomic sequences of strains A1 and B1 have been deposited in the GenBank/EMBL/DDBJ nucleotide sequence databases under accession codes AP014568 (strain A1), AP014569 (chromosome of strain B1) and AP014570 (plasmid in strain B1). Contig sequences corresponding to the genome of strain H1 have been deposited in the GenBank/EMBL/DDBJ nucleotide sequence databases under accession codes BAWN01000001 to BAWN01000094 . How to cite this article: Suzuki, S. et al. Physiological and genomic features of highly alkaliphilic hydrogen-utilizing Betaproteobacteria from a continental serpentinizing site. Nat. Commun. 5:3900 doi: 10.1038/ncomms4900 (2014).